Mesozoic retroposons reveal parrots as the closest living relatives of passerine birds The relationships of passerines (such as the well-studied zebra finch) with non-passerine birds is one of the great enigmas of avian phylogenetic research, because decades of extensive morphological and molecular studies yielded highly inconsistent results between and within data sets. Here we show the first application of the virtually homoplasy-free retroposon insertions to this controversy. Our study examined ~200,000 retroposon-containing loci from various avian genomes and retrieved 51 markers resolving early bird phylogeny. Among these, we obtained statistically significant evidence that parrots are the closest and falcons the second-closest relatives of passerines, together constituting the Psittacopasserae and the Eufalconimorphae, respectively. Our new and robust phylogenetic framework has substantial implications for the interpretation of various conclusions drawn from passerines as model organisms. This includes insights of relevance to human neuroscience, as vocal learning (that is, birdsong) probably evolved in the psittacopasseran ancestor, >30 million years earlier than previously assumed. Birds are important model organisms in many fields [1] , [2] , but ever since the time of Darwin, numerous attempts to reconstruct their phylogenetic relationships have yielded at least as many controversies [3] , [4] , [5] , [6] , [7] , [8] , [9] , [10] , [11] , [12] , [13] . In recent years, however, some morphological [3] , [4] and most molecular studies [7] , [8] , [9] , [10] , [11] , [12] , [13] have found congruence regarding the earliest chapters of bird evolution [14] . The root of extant birds lies between Palaeognathae (ratites and tinamous) and Neognathae, the latter comprising Galloanserae (chicken and ducks) and Neoaves (all remaining birds). Despite immense efforts, most of the basal relationships among Neoaves remain unsolved. This includes one issue of great interdisciplinary relevance [1] , [2] : the discovery of the putative sister group of passerines (>50% of all birds species, including all songbirds), one of the most-studied groups of animals [2] . Morphological studies indicated a close affinity either to woodpeckers [4] and rollers [3] or to cuckoos [5] , whereas a more basal position among Neoaves was suggested by DNA hybridization data [6] . On the other hand, nucleotide sequences of mitochondrial genomes placed passerines as the sister group to all remaining Neoaves [7] , [10] , to a woodpecker/roller/trogon clade [8] or to cuckoos [9] , whereas nuclear sequence analyses proposed a relation to woodpeckers and rollers [11] or to parrots [13] , falcons and seriemas [12] . A promising approach to overcome the present phylogenetic ambiguities is the use of retroposon insertions. Retroposons, jumping genetic elements that copy via RNA intermediates and insert nearly randomly anywhere in the genome (although some biases of insertion and retention have been proposed [15] ), provide (by inheritance) virtually homoplasy-free evidence of relatedness [16] that is detectable for more than 100 million years. Because parallel insertions or exact excisions are highly unlikely [16] , presence/absence patterns of retroposons at orthologous genomic loci are powerful, clear-cut phylogenetic markers capable of resolving long-standing uncertainties [17] , [18] , [19] , [20] . In this study, we present an improved resolution of bird evolution using retroposon insertions, a marker system that rarely undergoes homoplasy and is fully independent from previous approaches (for example, morphology, DNA hybridization or nucleotide sequence analyses). We provide the first statistically significant phylogenetic evidence for the early branching events in the avian tree of life, including the identification of the so far enigmatic sister group of passerines. Additionally, we reconstruct the chronological impact of retroposons on the avian genome during the Mesozoic Era of bird evolution. Reconstructing the avian tree of life using retroposon insertions From the over 200,000 retroposed elements (REs) present in the chicken and zebra finch genomes [1] , we selected the two most numerous fractions (>97% of all REs [1] ), namely, both the chicken repeat 1 (CR1) family of long interspersed elements (LINEs) and the long terminal repeat elements (LTRs) of endogenous retroviruses. Utilizing three different search strategies (Methods), we extracted 131 CR1 and 75 LTR loci that were experimentally tested via high-throughput PCR, leading to the identification of 51 phylogenetically informative markers. For each marker, representatives of the key avian lineages [13] , [14] were sampled, sequenced and aligned using standard procedures [21] . To measure the strength of support for all recovered branches, we calculated P values using the Waddell et al .' [22] likelihood ratio test for retroposon data. Thus, statistically significant retroposon evidence ( P <0.05) is reached with three conflict-free markers ( P =0.0370, (3 0 0)). Because of the mentioned strength and clearness of retroposon markers, our resultant maximum parsimony-based phylogenetic tree ( Fig. 1 , branches A–L) is effectively a maximum likelihood estimation [23] . 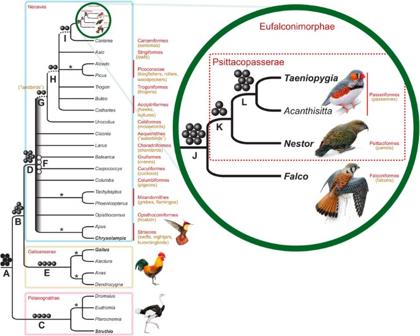Figure 1: Retroposon evidence for the early branching events in the avian tree of life. The tree topology is derived from our presence/absence matrix (Supplementary Table S1;Supplementary Software) utilizing maximum parsimony and considering representatives of the key avian lineages13,14. Black filled circles (branch A) are bird-specific retroposon insertions (exhibiting a 6-nt deletion that is found in some avian CR1s, but absent in all other avian and reptilian CR1s), and dark grey balls represent retroposon presence/absence markers that are congruent with one another. Light grey balls on grey gradient (label F) are retroposon markers that were probably inserted at the very beginning of the neoavian radiation and were subjected to incomplete lineage sorting of retroposon dimorphisms, as they exhibit presence/absence patterns that are incongruent with one another and with some of the retroposon markers on the dashed branches. Nodes without retroposon support are not collapsed (but highlighted by asterisks) if they received very strong support in nucleotide sequence analyses12,13,14. Higher-ranking taxa are in red letters (English terms in orange letters and parentheses), including the new taxa Eufalconimorphae (falcons+parrots+passerines) and Psittacopasserae (parrots+passerines), and some recently introduced superordinal groupings14,53,54. Bird names in bold letters belong to the nearest bird icon. Figure 1: Retroposon evidence for the early branching events in the avian tree of life. The tree topology is derived from our presence/absence matrix ( Supplementary Table S1 ; Supplementary Software ) utilizing maximum parsimony and considering representatives of the key avian lineages [13] , [14] . Black filled circles (branch A) are bird-specific retroposon insertions (exhibiting a 6-nt deletion that is found in some avian CR1s, but absent in all other avian and reptilian CR1s), and dark grey balls represent retroposon presence/absence markers that are congruent with one another. Light grey balls on grey gradient (label F) are retroposon markers that were probably inserted at the very beginning of the neoavian radiation and were subjected to incomplete lineage sorting of retroposon dimorphisms, as they exhibit presence/absence patterns that are incongruent with one another and with some of the retroposon markers on the dashed branches. Nodes without retroposon support are not collapsed (but highlighted by asterisks) if they received very strong support in nucleotide sequence analyses [12] , [13] , [14] . Higher-ranking taxa are in red letters (English terms in orange letters and parentheses), including the new taxa Eufalconimorphae (falcons+parrots+passerines) and Psittacopasserae (parrots+passerines), and some recently introduced superordinal groupings [14] , [53] , [54] . Bird names in bold letters belong to the nearest bird icon. Full size image Resolving early bird phylogeny Our retroposon markers are located on 14 different chromosomes, significantly clarifying more than the well-established [3] , [4] , [7] , [8] , [9] , [10] , [11] , [12] , [13] , [14] avian relationships. We obtained six retroposon insertions that are shared among paleognaths and neognaths, corroborating the monophyly of extant birds ( Fig. 1 , branch A). These retroposon insertions feature a unique, diagnostic deletion present only in some avian CR1 elements (subtypes CR1-Y and CR1-Z; this deletion is absent in crocodilian and all other avian CR1 elements), and can therefore be regarded as bird-specific REs ( Supplementary Fig. S1 ). Additionally, the root of living birds is located between the significantly supported Neognathae ( Fig. 1 , branch B; five REs, P =0.0041, (5 0 0), likelihood ratio test [22] ) and Palaeognathae ( Fig. 1 , branch C; four REs, P =0.0123, (4 0 0), likelihood ratio test [22] ). Significant support was also found for the monophyly of Neoaves ( Fig. 1 , branch D; six REs, P =0.0014, (6 0 0), likelihood ratio test [22] ), Galloanserae ( Fig. 1 , branch E; four REs, P =0.0123, (4 0 0), likelihood ratio test [22] ) and Passeriformes ( Fig. 1 , branch L; six REs, P =0.0014, (6 0 0), likelihood ratio test [22] ). Resolving the neoavian radiation Within the hitherto largely unresolved [7] , [8] , [9] , [10] , [11] , [12] , [13] , [14] radiation of Neoaves, we obtained four markers whose insertion patterns seem inconsistent with one another ( Fig. 1 , label F; Supplementary Fig. S2 ; Supplementary Table S1 ). As CR1 and LTR retroposons exhibit no or very short (<6 bp) target site duplications, exact excisions as proposed for primate Alu short interspersed elements [24] cannot have occurred [25] . Because of the nearly 1.2 billion [1] potential insertion sites in the avian genome, parallel insertions (featuring exactly the same target site, retroposon type, orientation and truncation) should be extremely rare. Therefore, the incongruent patterns among the four retroposon insertions are most likely a result of incomplete lineage sorting (leading to hemiplasy) [26] of retroposon presence/absence dimorphisms that persisted during the very beginning of the neoavian radiation and were randomly fixed (that is, one of the two alleles was lost) in each of the descendant lineages ( Supplementary Fig. S2 ). This complex evolutionary phenomenon was previously revealed by retroposons (for example, in the rapid radiations of cichlid fishes [27] and placental mammals [17] , [20] ) and is a further indication that the earliest period of the rapid radiation of Neoaves is a putative polytomy [28] . The remaining retroposon evidence within Neoaves exhibits no incongruent presence/absence patterns. We recovered the previously reported [12] , [13] 'landbird' assemblage ( Fig. 1 , branch G; two REs), a novel clade consisting of all 'landbirds' to the exclusion of mousebirds ( Fig. 1 , branch H; two REs) and a close affinity [12] , [13] among seriemas, falcons, parrots and passerines ( Fig. 1 , branch I; two REs). Statistical testing [22] of the support for these three branches is not applicable, as some of the above incongruent presence/absence patterns are also inconsistent to these ( Supplementary Fig. S2 ; Supplementary Table S1 ). Unexpectedly, we obtained a wealth of conflict-free retroposon markers for two branches that were previously proposed by the Hackett et al . [13] study of nuclear intronic sequences, and which received relatively moderate bootstrap support in their study. Seven retroposon insertions are exclusively present in falcons, parrots and passerines, but absent in hawks, woodpeckers and other 'landbirds' ( Fig. 1 , branch J; seven REs, P =0.0005, (7 0 0), likelihood ratio test [22] ); we therefore suggest the new name Eufalconimorphae (true Falconimorphae) for this significantly supported monophylum. Most strikingly, the shared presence of three retroposon insertions solely in parrots and passerines ( Fig. 1 , branch K; three REs, P =0.0370, (3 0 0), likelihood ratio test [22] ; see also Fig. 2 for sequence alignments) provides statistically significant evidence of parrots as the living sister group of the Passeriformes. To make this new phylogenetic resolution easily comprehensible, we propose the new name Psittacopasserae (parrots and passerines). It is worth noting that with this evidence, for the first time, passerines can be confidently placed within the avian tree of life. 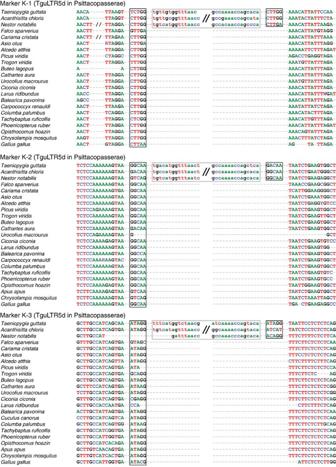Figure 2: Alignment of presence/absence regions of three monophyly markers for Psittacopasserae. Potential target site duplications (direct repeats) are in black boxes, 5′ and 3′ ends of the retroposon insertions are shown in lower case letters in grey boxes. Figure 2: Alignment of presence/absence regions of three monophyly markers for Psittacopasserae. Potential target site duplications (direct repeats) are in black boxes, 5′ and 3′ ends of the retroposon insertions are shown in lower case letters in grey boxes. Full size image Although our exhaustive zebra finch-based retroposon screening did not detect any evidence for incomplete lineage sorting within Eufalconimorphae, we cannot completely exclude the possibility of its occurrence in this part of the neoavian tree. Considering this, we expect that, once the genome sequence of a parrot or a falcon is available, parrot- or falcon-based retroposon screenings will permit an even stronger resolution of this issue and a reevaluation of the conflict-free support for Psittacopasserae reported here. Reconstructing the chronology of Mesozoic retroposon activity In addition to resolving phylogenetic controversies, our markers enabled us to reconstruct the temporal retroposon impact on the avian genome during early bird phylogeny via the comparison of these experimentally verified insertion events with computational estimates of retroposon activity. To determine a computational chronology of retroposon activities, 995 nested retroposons (retroposons that inserted into other retroposons) were extracted from the zebra finch genome and their coordinates were implemented in the transposition in transposition (TinT) model [25] , [29] . Because the insertion of a younger (active) RE subtype into an older (inactive) RE can be expected to occur more likely than the opposite situation, the genome-wide quantitative distribution of different subtypes of retroposons nested within other RE subtypes enables a reliable estimation of relative retroposon activity periods [29] . As some RE subtypes were active during relatively short periods, it is possible to plot the resulting TinT pattern against a chronogram of molecular divergence times [30] , yielding a congruent estimate of retroposon successions during the Mesozoic evolution of birds [12] , [30] ( Fig. 3 ). For instance, both approaches indicate that during the shared evolutionary history of the chicken and zebra finch (in the lineage leading to Aves and Neognathae), several retroposons (CR1-Y2_Aves, CR1-Y1_Aves and TguLTR5e) were active (see Supplementary Fig. S3 for a TinT pattern of the chicken genome). Subsequently, other REs (CR1-E_Pass, CR1-J2_Pass, TguLTR5a and TguLTR5d) were active in the ancestor of Neoaves and within the neoavian radiation. Considering that most of the identified retroposon markers that were inserted during the neoavian radiation are LTRs (including all evidence for Eufalconimorphae and Psittacopasserae), we assume that this period of extensive and accelerated speciation events was accompanied by an increased activity of endogenous retroviruses. This conclusion coincides with the observation that the zebra finch genome harbours about three times as many LTRs as the chicken genome [1] . Moreover, our zebra finch TinT pattern indicates that the greatest retroposon diversity was present during and bordering the neoavian radiation, including many different short-lived subtypes of REs. On the basis of these insights, future retroposon studies can easily select the REs that were active during an evolutionary chapter of interest to resolve the remaining uncertainties regarding the earliest divergences within Neoaves. 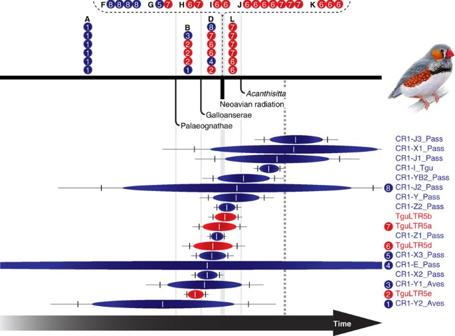Figure 3: Chronology of Mesozoic retroposon activity in the zebra finch genome. Computational estimates of activity periods (normal distributions displayed as ovals29) of selected retroposon subtypes were calculated using the TinT model25,29and plotted on a simplified chronogram30(black lines) using the experimentally verified retroposon insertion events (numbered blue or red balls, numbers indicate the respective retroposon subtype) ofFigure 1as temporal landmarks. Single capital letters correspond to the branch labels ofFigure 1(A, Aves; B, Neognathae; D, Neoaves; F, incongruent markers; G, 'landbirds'; H, 'landbirds' without mousebirds; I, Eufalconimorphae+seriemas; J, Eufalconimorphae; K, Psittacopasserae; L, Passeriformes). CR1 retroposons are highlighted in blue and LTR retroposons are shown in red. The dashed bracket consists of retroposon markers that were inserted during the neoavian radiation; the grey dashed vertical line indicates the estimated end of the Mesozoic Era at the Cretaceous/Tertiary boundary30. We note that the exceptionally long TinT activity range of the CR1-E_Pass element (no. 4) is most probably an overestimation because of CR1 subfamily misidentification, as only a few diagnostic nucleotides distinguish this retroposon from other CR1 subfamilies. Figure 3: Chronology of Mesozoic retroposon activity in the zebra finch genome. Computational estimates of activity periods (normal distributions displayed as ovals [29] ) of selected retroposon subtypes were calculated using the TinT model [25] , [29] and plotted on a simplified chronogram [30] (black lines) using the experimentally verified retroposon insertion events (numbered blue or red balls, numbers indicate the respective retroposon subtype) of Figure 1 as temporal landmarks. Single capital letters correspond to the branch labels of Figure 1 (A, Aves; B, Neognathae; D, Neoaves; F, incongruent markers; G, 'landbirds'; H, 'landbirds' without mousebirds; I, Eufalconimorphae+seriemas; J, Eufalconimorphae; K, Psittacopasserae; L, Passeriformes). CR1 retroposons are highlighted in blue and LTR retroposons are shown in red. The dashed bracket consists of retroposon markers that were inserted during the neoavian radiation; the grey dashed vertical line indicates the estimated end of the Mesozoic Era at the Cretaceous/Tertiary boundary [30] . We note that the exceptionally long TinT activity range of the CR1-E_Pass element (no. 4) is most probably an overestimation because of CR1 subfamily misidentification, as only a few diagnostic nucleotides distinguish this retroposon from other CR1 subfamilies. Full size image Our results have far reaching implications from more than an ornithological point of view. In addition to the reconstruction of speciation events in early bird phylogeny, we have established a calibrated chronology of retroposon activity during the Mesozoic Era of bird evolution. We identified retroposons that were inserted at the very beginning of the neoavian radiation and were probably subjected to incomplete lineage sorting, a phenomenon that likely accounts for some of the incongruent results from sequence-based phylogenies. Retroposons constitute unique tools for understanding such complex and otherwise irresolvable evolutionary scenarios [27] . Furthermore, we have determined a statistically significant resolution of a later part of the neoavian radiation, namely, the sister group relationship of passerines and parrots (Psittacopasserae) and their mutual affinity to falcons (Eufalconimorphae). Our retroposon evidence can serve as a robust prior hypothesis for future studies focusing on these bird taxa. As such, parrots and passerines not only share the ability to learn vocalization [2] , but also have a direct common ancestor. Although hummingbirds are also vocal learners [31] , our phylogeny indicates that they are only distantly related to Psittacopasserae; therefore it is most parsimonious to assume that their vocal learning capability evolved after the divergence of hummingbirds and swifts ( Fig. 4 ). Nevertheless, the phylogenetic resolution of Psittacopasserae raises the question as to what extent the striking neuroanatomical and gene expression parallels [2] (for example, the anterior-medial vocal pathway [32] ) between parrots and oscine passerines (songbirds) are homologous and thus evolved in their shared ancestor ( Fig. 4 ). Behavioural and neuroanatomical data on 'non-oscine' passerines (Suboscines and Acanthisittidae) is scarce [33] and, to our knowledge [34] , limited to New World Suboscines, suggesting that some representatives do not learn vocalizations (that is, Tyrannidae [35] , [36] , [37] ), whereas others possibly do (that is, the earlier-branching [38] Cotingidae [33] and Pipridae [39] ). Thus, to assume that vocal learning evolved in the psittacopasseran ancestor (with a secondary loss in at least one lineage of suboscine passerines) seems more parsimonious than hypothesizing four independent evolutions of vocal learning within Psittacopasserae. Accordingly, the emergence of vocal learning of songbirds would have happened at least 30 million years [30] earlier than evident from the previous assumption of the independent evolution of cerebral vocal nuclei [40] in parrots and in (oscine) passerines. Thorough reevaluation of this issue will impact various conclusions drawn from passerines and might thereby change our current understanding of the evolution of vocal learning in general. 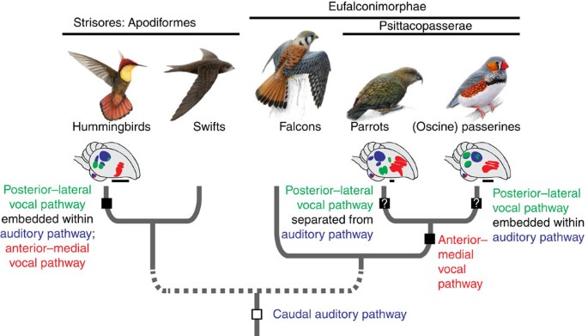Figure 4: Evolution of vocal learning in birds. Schematic brain drawings (adapted from Jarviset al.31) depict the hearing- and vocalizing-induced ZENK transcription factor expressions in hummingbirds, budgerigars (parrot representatives) and songbirds (passerine representatives). Our robust phylogenetic framework implies that some traits associated with vocal learning (for example, the anterior–medial vocal pathway (red)) are potentially homologous and thus evolved as an autapomorphic trait (black square) in the psittacopasseran ancestor, but also independently in the distantly related ancestor of hummingbirds (dashed lines indicate that several neoavian lineages are not shown). Neuroanatomical studies on early branching passerines (that is, Suboscines and Acanthisittidae) are necessary to infer that the posterior–lateral vocal pathway (green, located at different brain regions in parrots and oscine passerines) is either homologous or evolved independently in the two lineages. The caudal auditory pathway (blue) is a plesiomorphic trait (white square) and was probably inherited from a common avian ancestor32. The putative location of the auditory pathway in falcons and swifts is not shown, as ZENK expression patterns have, to our knowledge, not yet been investigated in these birds. Scale bar, 2 mm. Figure 4: Evolution of vocal learning in birds. Schematic brain drawings (adapted from Jarvis et al . [31] ) depict the hearing- and vocalizing-induced ZENK transcription factor expressions in hummingbirds, budgerigars (parrot representatives) and songbirds (passerine representatives). Our robust phylogenetic framework implies that some traits associated with vocal learning (for example, the anterior–medial vocal pathway (red)) are potentially homologous and thus evolved as an autapomorphic trait (black square) in the psittacopasseran ancestor, but also independently in the distantly related ancestor of hummingbirds (dashed lines indicate that several neoavian lineages are not shown). Neuroanatomical studies on early branching passerines (that is, Suboscines and Acanthisittidae) are necessary to infer that the posterior–lateral vocal pathway (green, located at different brain regions in parrots and oscine passerines) is either homologous or evolved independently in the two lineages. The caudal auditory pathway (blue) is a plesiomorphic trait (white square) and was probably inherited from a common avian ancestor [32] . The putative location of the auditory pathway in falcons and swifts is not shown, as ZENK expression patterns have, to our knowledge, not yet been investigated in these birds. Scale bar, 2 mm. Full size image General approach We used three different search strategies to computationally screen over 200,000 REs present in the chicken and zebra finch genomes (see Supplementary Table S1 for information on the contribution of each strategy to the 51 phylogenetically informative markers). On the basis of their suitability for cross-species PCR amplification (that is, only retroposon insertions situated in well-conserved intronic or intergenic regions smaller than 1.5 kb were considered), we identified 131 CR1 and 75 LTR candidate RE-containing loci. These loci were then experimentally screened in a reduced taxon sampling (comprising Nestor , Falco , Picus , Buteo , Ciconia and Columba for zebra finch REs; in the case of chicken and emu REs, the reduced taxon sampling consisted of the representatives of Galloanserae and Palaeognathae), revealing our 51 phylogenetically informative markers. In silico screening Initially, (first strategy; a) genomic three-way alignments (comprising emu, chicken, and zebra finch) were compiled by MAFFT [41] (FFT-NS-2, version 6, http://mafft.cbrc.jp/alignment/server/index.html ) using ~2.55 million bp of emu genomic contigs available in GenBank ( http://www.ncbi.nlm.nih.gov/Genbank/ ) and the corresponding regions in the chicken and zebra finch genomes (assemblies galGal3 and taeGut1 in Genome Browser [42] , http://genome.ucsc.edu/cgi-bin/hgBlat ). REs were annotated using CENSOR ( http://www.girinst.org/censor/index.php ), and retroposon insertion loci situated in well-conserved intronic or intergenic regions were chosen for primer generation. To identify additional candidate loci (first strategy; b), all avian sequences available in GenBank were screened for REs and (if a retroposon was present) aligned to the corresponding regions in the chicken and zebra finch genomes using MAFFT (E-INS-I, version 6). Second strategy; based on the insights gained by strategy I into the phylogenetic informativeness of representatives of certain CR1 and LTR subfamilies for our phylogenetic questions of interest, whole-genome in silico screenings for selected retroposons were conducted. This was done by extracting retroposon insertions including their flanking sequences (1 kb of each flank) from chicken or zebra finch genomes and BLAST screening these against chicken annotated unique exonic sequences to obtain well-conserved loci (<1.5 kb). Alternatively, retroposon consensus sequences from Repbase ( http://www.girinst.org/repbase/index.html ) were BLAT [43] screened against chicken or zebra finch genomes and well-conserved loci in introns (of any size) or intergenic regions were chosen for primer generation. Third strategy; a CR1-enriched retroposon library of emu genomic DNA was constructed via a protocol utilizing digestion and circularization of genomic DNA and subsequent inverse PCR [44] . A total of 242 clones were sequenced and BLAT screened against chicken and zebra finch genomes to find CR1 insertions (situated in well-conserved regions) specific to the lineage leading to the emu and suitable for experimental presence/absence screening. Taxon sampling Our whole taxon sampling (voucher numbers of the samples in the LWL-DNA- und Gewebearchiv of the Museum für Naturkunde Münster are specified) consisted of representatives of the key lineages [13] , [14] within Palaeognathae ( Struthio camelus (LWL00446), Pterocnemia pennata (LWL00447), Eudromia elegans (LWL00448), Dromaius novaehollandiae (LWL00449)), Galloanserae ( Dendrocygna viduata (LWL00450), Anas crecca (LWL00451), Alectura lathami (LWL00452), Gallus gallus (LWL00453)) and Neoaves ( Chrysolampis mosquitus (LWL00458), Apus apus (LWL00459), Opisthocomus hoazin (LWL00457), Phoenicopterus ruber roseus (LWL00454), Tachybaptus ruficollis (LWL00455)/ Podiceps cristatus (LWL00456), Columba palumbus (LWL00408), Carpococcyx renauldi (LWL00460)/ Cuculus canorus (LWL00461), Balearica pavonina (LWL00462), Larus ridibundus (LWL00463), Ciconia ciconia (LWL00464)/ C. boyciana , Urocolius macrourus (LWL00465), Cathartes aura (LWL00466)/ Gymnogyps californianus , Buteo lagopus (LWL00467)/ Gyps fulvus (LWL00468), Trogon viridis (LWL00469), Picus viridis (LWL00470), Alcedo atthis (LWL00105), Asio otus (LWL00417), Cariama cristata (LWL00474), Falco sparverius (LWL00471), Nestor notabilis (LWL00472), Acanthisitta chloris (LWL00475) and Taeniopygia guttata (LWL00473)). Species identity was confirmed by direct sequencing of a fragment of the mitochondrial ND2 gene using the published primers L5216+H6313 (courtesy of Michael D. Sorenson, Boston University) listed in Supplementary Table S2 , and subsequent BLAST screening against GenBank's nucleotide collection and our own unpublished mitochondrial sequences. If no sequence or only the sequence of a closely related species was publicly available, we deposited the respective new ND2 sequence in GenBank. In vitro screening The marker candidates selected using our three in silico screening strategies were experimentally tested for their phylogenetic informativeness (see Supplementary Table S1 for presence/absence patterns of the 51 phylogenetically informative markers) using a taxon sampling that is essential for a phylogenetic conclusion. Genomic DNA was isolated from blood or muscle tissue using conventional phenol–chloroform extraction, whereas contour feathers were processed either via the QIAamp DNA Micro kit (Qiagen) using a modified protocol [45] or using a rapid simple alkaline extraction [46] . Each 25-μl PCR reaction contained 0.5 U ThermoPrime Taq DNA Polymerase (ABgene), 75 mM Tris–HCl, pH 8.8, 20 mM (NH 4 ) 2 SO 4 , 0.01% (v/v) Tween 20, 2.5 mM MgCl 2 , 0.1 mM of each deoxyribonucleotide triphosphate, 10 pmol of each primer (see Supplementary Table S2 for primer sequences) and >5 ng of genomic DNA. PCRs were carried out using the touchdown PCR strategy; 2 min at 94 °C were followed by 10 cycles of 30 s at 94 °C, 30 s at 55 °C (decreasing by 1 °C per cycle) and 80 s at 72 °C. The final 26 cycles of 30 s at 94 °C, 30 s at 45 °C and 80 s at 72 °C were followed by 120 s at 72 °C. Subsequent to agarose gel electrophoresis, all PCR products were immediately purified or excised from agarose gels and then purified. Sequencing of the samples was conducted either directly using the specific PCR primers or indirectly using standard M13 forward and reverse primers after ligation into the pDrive Cloning Vector (Qiagen) and electroporation into TOP10 cells (Invitrogen). RE analysis All nucleotide sequences were deposited in GenBank (accession numbers JF915895-JF916445 ). To complete our taxon sampling, we also used previously published sequences available in Genome Browser (assemblies galGal3 [47] and taeGut1 [1] ) and GenBank (accession numbers AB112956 , AB235826 , AB235829 , AC153776 , AC158282 , AC158284-AC158286 , AC160232 , AF525979 , AF525980 , DP000685 , DP000802 , JF279549-JF279555 , JF279558–JF279573 and JF279576–JF279590 ). Some of the sequence data [48] , [49] , [50] (emu BAC sequences AC153776, AC158282, AC158284–AC158286, AC160232, DP000685 and DP000802; alligator BAC sequences DP000795 and DP000976) were generated by the National Institutes of Health Intramural Sequencing Center ( http://www.nisc.nih.gov ). The lizard genome sequence (assembly anoCar1 in Genome Browser) was generated by the Broad Institute ( http://www.broadinstitute.org ). All sequences of each marker were first automatically aligned using MAFFT (E-INS-I, version 6) and then manually realigned (see Supplementary Data for 51 full sequence alignments). Each alignment was carefully inspected and the retroposon insertion considered a phylogenetically informative marker if, in all species sharing this RE, it featured an identical orthologous genomic insertion point (target site), identical RE orientation, identical RE subtype, identical target site duplications (direct repeats, if present) and a clear absence in other species. Candidate markers exhibiting an RE flanked by >10 bp of nearly identical, low-complexity sequences were excluded from the analysis to minimize the possibility of inconsistencies caused by precise RE excision as reported by van de Lagemaat et al . [24] In the case of CR1 retroposon insertions shared among all the investigated bird lineages (markers A-1 to A-6), we initially aligned the avian retroposon flanks to the corresponding BAC sequences of the alligator available in GenBank (DP000795 and DP000976). Because of the ~220 million years of bird/crocodilian sequence divergence [51] , a classical presence/absence situation could not be ascertained. Although CR1 elements are also found in the genomes of other non-mammalian amniotes [48] , [49] , [50] , we consider these retroposon insertions to be suitable markers for the monophyly of birds, because each of them exhibits a diagnostic 6-nt deletion that is only present in a few bird-specific CR1 subtypes (that is, CR1-Y and CR1-Z) but not in CR1 elements of other amniotes (that is, all BLAST and BLAT search hits of avian CR1 against available genome or BAC sequences of alligator, lizard, turtle, platypus and human were inspected by eye; see Supplementary Fig. S1 for a structural comparison of the well-conserved terminal regions [52] of amniote CR1 retroposons including lineage-specific diagnostic insertions or deletions). The majority-rule consensus sequences of the previously unrecognized CR1 subtypes 'ALL-LINEa', 'ALL-LINEb' and 'ANO-LINE' were derived from 17, 25 and 10 BLAST hits, respectively. On the basis of the presence/absence matrix of our 51 phylogenetically informative markers ( Supplementary Table S1 ), our phylogenetic tree was drawn by hand considering maximum parsimony and independently verified by a maximum parsimony analysis of a 1/0-coded version of our presence/absence matrix ( Supplementary Software ) in PAUP*(version 4.0b10; using the irrev.up option of character transformation, heuristic search with 1000 random sequence additions, and TBR branch swapping). This yielded one strict consensus parsimony tree ( Fig. 1 , consistency index=0.895 and tree length=57) derived from 577 equally parsimonious trees. TinT analysis To determine a chronology of retroposon activity periods, we used the web-based TinT application [29] ( http://www.compgen.uni-muenster.de/tools/tint/ ). As input data, the precomputed RepeatMasker files (hosted on the server) from chicken or zebra finch were selected. Only the retroposon subtypes present in the respective figures (see Fig. 3 for the zebra finch TinT of 995 nested REs or Supplementary Fig. S3 for the chicken TinT of 2355 nested REs) were included in the analysis (but note that, in the case of the zebra finch TinT, the retroposons CR1-YB1_Tgu and TguLTR5c were added to the analysis but excluded from Fig. 3 ) using default parameters. The resultant graph of normal distributions of retroposon activity (ovals represent 75%, vertical lines 95% and horizontal lines 99% of the probable activity period) was plotted on a simplified chronogram [30] using the experimentally verified retroposon insertions of Figure 1 as calibration points (for example, the succession of TguLTR5e to TguLTR5d activity in the zebra finch ancestor's genome after the divergence of Galloanserae and Neoaves). For this purpose, we considered the chronogram by Pereira and Baker [30] to be most suitable, as it includes molecular divergence times for the Crocodylia/Aves split, the Palaeognathae/Neognathae split, the neoavian radiation, and the Acanthisitta /oscine Passeriformes split (other analyses of molecular divergence times [8] , [12] have only investigated a few of these dates). Accession codes: The nucleotide sequences have been deposited in GenBank database under accession numbers JF915895–JF916445 . How to cite this article: Suh, A. et al . Mesozoic retroposons reveal parrots as the closest living relatives of passerine birds. Nat. Commun. 2:443 doi: 10.1038/ncomms1448 (2011).